Photonic Aharonov–Bohm effect in photon–phonon interactions The Aharonov–Bohm effect is one of the most intriguing phenomena in both classical and quantum physics, and associates with a number of important and fundamental issues in quantum mechanics. The Aharonov–Bohm effects of charged particles have been experimentally demonstrated and found applications in various fields. Recently, attention has also focused on the Aharonov–Bohm effect for neutral particles, such as photons. Here we propose to utilize the photon–phonon interactions to demonstrate that photonic Aharonov–Bohm effects do exist for photons. By introducing nonreciprocal phases for photons, we observe experimentally a gauge potential for photons in the visible range based on the photon–phonon interactions in acousto-optic crystals, and demonstrate the photonic Aharonov–Bohm effect. The results presented here point to new possibilities to control and manipulate photons by designing an effective gauge potential. The Aharonov–Bohm (AB) effect is a quantum mechanical phenomenon in which the phase of a charged particle is affected by the vector potential of an electromagnetic field ( E , B ) even when both the magnetic field B and electric field E vanish on the trajectory of the particle [1] . The AB effect has been experimentally demonstrated with charged particles, such as electrons [2] , and has found applications in various fields, including quantum interference at the single-molecule level [3] , [4] , characterizations of the micro and nanostructures and materials [5] , [6] , [7] , [8] , and matter wave investigations [9] . Recent research has started to ask if any AB effects exist for neutral particles, such as photons. In Fang et al. [10] , [11] it was theoretically proposed that when the refractive index of a photonic system is modulated, the phase of the refractive index modulation represents a gauge potential for photons and is nonreciprocal. Also a proper choice of the modulation phase can be used to induce a photonic AB effect. This proposal has been demonstrated in the radio-wave and infrared frequency ranges [12] , [13] . Such AB effect is also closely related to recent efforts seeking to achieve dynamically induced nonreciprocity without the use of magneto-optical effects [14] , [15] , [16] . Here we propose theoretically and demonstrate experimentally in the visible wavelength range that the photonic AB effect can arise through the photon–phonon interaction within acousto-optic crystals, which introduce nonreciprocal phases to the photons in the visible range travelling in two opposite directions. The experiment carried out in this work is classical, but the nonreciprocal phase induced by the photon–phonon interaction should persist at the single-photon level, where novel quantum interference effect can arise. The results presented here may find applications in photonics, providing new mechanisms to control and manipulate photons. Electronic AB effect In the experiment demonstrating the electronic AB effect, a coherent electron beam is split into two, which recombine after propagating along two different paths that enclose a magnetic field. The magnetic field is spatially localized between the two paths, such that both the E and B fields vanish on the two paths. In spite of the lack of B fields along the paths that the electron takes, one nevertheless observes that, after the beams recombine, the electron probability amplitude oscillates in a sinusoidal manner as the flux Φ M of the applied magnetic field is varied. The AB effect demonstrates the fundamental role that the vector potential plays in electron physics. According to quantum mechanics, an electron propagating in the presence of a vector potential A acquires a phase shift (that is, in addition to the regular propagation phase). This additional phase is nonreciprocal: reversing the propagation direction of the electron changes its sign. Hence the presence of the vector potential can break the time-reversal symmetry for electrons. Also, this phase depends on the gauge choice; for an open propagation pathway this phase is not uniquely defined and hence is not in itself an observable. However, the phase difference between two different pathways is observable and depends linearly on the magnetic flux that the two pathways enclose. Such a phase difference is known as the magnetic AB phase shift. Examining equation (2), we see that for neutral particles, such as photons, no magnetic AB phase shifts exist as e =0. There is therefore no naturally occurring gauge potential for photons. Photonic AB effect in photon–phonon interaction It has been shown in Fang et al. [10] , [11] that photonic transitions between two photonic modes |1› and |2› can be used to achieve an effective gauge potential for photons. Here we propose the use of the interactions between photons and phonons for this purpose. The photon–phonon interaction plays an important role in modern physics and device applications [17] , [18] . Here we realize photonic transition in photon–phonon interactions and experimentally demonstrate a gauge potential for photons, and a photonic AB effect, based on the photon–phonon interaction. With the acousto-optic effect, photons can be scattered by phonons in a crystal [19] , [20] . As shown in Fig. 1 , here we consider a scattering process where an incident photon in an incident beam as denoted by mode |1›, with an angular frequency ω 1 and a wavevector k 1 , interacts with a phonon of an angular frequency Ω and a wavevector q . The photon–phonon interaction will generate a photon in a diffracted beam as denoted by a different mode |2›, which has a different frequency ω 2 and a wavevector k 2 . This process satisfies the conservations of energy and momentum, that is, ħω 2 = ħω 1 ± ħΩ and ħ k 2 = ħ k 1 ± ħ q , from which the Doppler frequency shift formula, ω 2 = ω 1 ± Ω , and the Bragg condition [21] , k 2 = k 1 ± q , follow. The plus and minus signs imply that the outgoing photon can either be upshifted or downshifted in frequency, and that photonic transitions between the two photonic modes |1› and |2› are reversible, depending on the configuration of the photon–phonon interaction. Another important feature of the photon–phonon interaction is that with appropriate design the outgoing photon can travel in a different path from the incoming photon, which is critical for spatially separating the scattered photons from unscattered ones to avoid possible interferences between the diffracted and undiffracted beams. 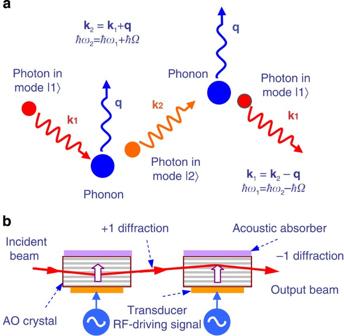Figure 1: Illustration of photon–phonon interactions in acousto-optic crystals. (a) Photon–phonon interactions. A photon in mode |1› interacts with a phonon, generating a photon in mode |2›, which interacts with another phonon. Through the cascaded photon–phonon interactions, photonic transitions from mode |1› to mode |2› and back to mode |1› are realized. Each stage of the photon–phonon interactions satisfies the Bragg condition and the conservations of energy and momentum. (b) Interactions of laser beams with acoustic waves within two acousto-optic (AO) crystals. The first-order diffracted beam from the first AO crystal is used as the input beam of the second AO crystal, and the minus first-order diffracted beam from the second AO crystal is selected as the output beam, therefore the frequency shifts from the two AO crystals cancel each other, but the phase difference between the two radio-frequency (RF)-driving signals of the two AO crystals is imprinted as a phase delay of the output beam. Figure 1: Illustration of photon–phonon interactions in acousto-optic crystals. ( a ) Photon–phonon interactions. A photon in mode |1› interacts with a phonon, generating a photon in mode |2›, which interacts with another phonon. Through the cascaded photon–phonon interactions, photonic transitions from mode |1› to mode |2› and back to mode |1› are realized. Each stage of the photon–phonon interactions satisfies the Bragg condition and the conservations of energy and momentum. ( b ) Interactions of laser beams with acoustic waves within two acousto-optic (AO) crystals. The first-order diffracted beam from the first AO crystal is used as the input beam of the second AO crystal, and the minus first-order diffracted beam from the second AO crystal is selected as the output beam, therefore the frequency shifts from the two AO crystals cancel each other, but the phase difference between the two radio-frequency (RF)-driving signals of the two AO crystals is imprinted as a phase delay of the output beam. Full size image We now consider the cascading of two photon–phonon scattering events, where a photon in mode |1› is transformed to mode |2› with a different frequency through the first photon–phonon interaction event. The photon is then subsequently converted back to mode |1› by a second photon–phonon scattering event. Such a cascading process was previously used to demonstrate an acousto-optic phase shifter [22] . We will show that such a cascade process induces a nonreciprocal phase and can be used to demonstrate the photonic AB effect. Our experimental set-up is schematically illustrated in Fig. 2 . To achieve two-stage photon–phonon interactions, two acousto-optic modulators (AOM), AOM1 and AOM2, are employed and arranged in a tandem manner ( Fig. 1b ). The operation of each AOM can be described by the coupled-wave method [18] . 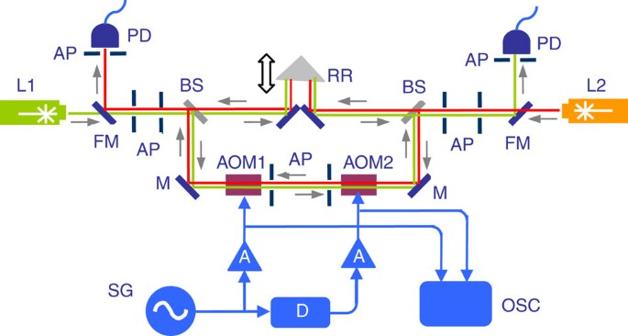Figure 2: Schematic of the experimental set-up for demonstrating photonic Aharonov–Bohm (AB) effect. Two acousto-optic modulators, AOM1 and AOM2, are arranged in a tandem manner to introduce nonreciprocal phases to the photons travelling in two opposite directions. Switching between two transmission directions is realized by flipping the two mirrors (FMs) in front of the lasers. Arrows are used for indicating the directions of the laser beams in the interferometer. L1 and L2, He–Ne lasers; PD, photo-detector; M, mirror; AP, aperture; SG, RF generator; A, RF amplifier; D, RF delay line; OSC, oscilloscope. For the first AOM, suppose that the electric field of the incident beam is Figure 2: Schematic of the experimental set-up for demonstrating photonic Aharonov–Bohm (AB) effect. Two acousto-optic modulators, AOM1 and AOM2, are arranged in a tandem manner to introduce nonreciprocal phases to the photons travelling in two opposite directions. Switching between two transmission directions is realized by flipping the two mirrors (FMs) in front of the lasers. Arrows are used for indicating the directions of the laser beams in the interferometer. L1 and L2, He–Ne lasers; PD, photo-detector; M, mirror; AP, aperture; SG, RF generator; A, RF amplifier; D, RF delay line; OSC, oscilloscope. Full size image and the field of the acoustic wave in the first acousto-optic crystal is where Ω is the angular frequency of the RF signal that drives the transducer. Inside the crystal, the density (and hence the refractive index) of the material is modulated by the acoustic wave. The refractive index modulation acts as a moving grating in the crystal (in an AOM device, the crystal is normally angle cut or an acoustic absorber is attached to the opposite end of the transducer to ensure a travelling wave is generated in the crystal, as shown in Fig. 1b ). The incident beam can be diffracted into either the +1 diffraction order with a frequency ω 2 = ω 1 + Ω , or the −1 diffraction order with a frequency ω 2 = ω 1 − Ω , depending on the direction of the incident beam to the acoustic wave, as determined by the Bragg condition. When the incident beam is against the propagation direction of the acoustic wave, as shown in Fig. 1b , the diffraction occurs in the +1 order resulting in a positive frequency shift. Therefore, at the exit of the first modulator, AOM1, the electric field of the diffracted beam becomes where ϕ 1 is a phase delay associated with the optical path from the entrance to the exit of AOM1. Notice that the phase of the acoustic wave, Φ 1 , is now imprinted as a phase of the diffracted beam. The diffraction beam generated by AOM1 enters the second modulator, AOM2, in which the field of the acoustic wave can be expressed as Note, in contrast with the first modulator (AOM1), AOM2 is arranged so that the incident beam is along the propagation direction of the acoustic wave. Therefore, the first-order diffracted beam generated by AOM2 acquires a negative frequency shift. As the two AOMs are driven by the signals with the same angular frequency Ω , the frequency shifts as generated by the two AOMs cancel. The electric field of the first-order diffracted beam of AOM2 can be expressed as where ϕ 2 is the total propagation phase delay accumulated as the photon propagates along optical path from the entrance of AOM1 to the exit of AOM2. As the photon–phonon interactions occurred in AOM1 and AOM2 are in opposite directions, we have k 3 =k 1 . Thus, the photons in mode |1› are converted to mode |2› on passing through the first AOM, and then the photons are converted back to mode |1› on passing through the second AOM. In this process, in addition to the propagation phase ϕ 2 , the photon acquires an additional phase shift Φ 1 – Φ 2 , which is the phase difference between the two acoustic waves. We now consider the time-reversed process, where a photon, injected from the right, passes through AOM2 first before entering AOM1. In this case, repeating the same derivation as above, we see that the photon picks up a phase delay of ϕ 2 + Φ 2 − Φ 1 . Notice that the sign change of the additional phase is related to the phases of the acoustic fields. The system response is therefore nonreciprocal. We argue that the phases of the acoustic fields, that is, Φ 1 and Φ 2 , impose a gauge potential for photons. As far as the photon is concerned, the phase of a single acoustic wave, for example, Φ 1 , is undetectable and hence represents a gauge degree of freedom, having exactly the same gauge ambiguity as the phase induced by a line integral of an electronic gauge potential along an open path as in Equation (1). The phase difference between the two AOMs, that is, Φ 1 − Φ 2 , on the other hand, is detectable in the interferometer set-up as shown in Fig. 2 . Moreover, reverting the propagation direction of the photons results in the change of the sign of this phase difference. Thus, this phase difference has exactly the same property as the AB phase shift of Equation (2). The interferometer set-up of Fig. 2 is used to detect such phase difference between the two propagation directions. Compared with the electronic AB interferometer, our set-up also detects the nonreciprocal phase shifts as induced by a gauge degree of freedom, therefore, the set-up here represents a photonic AB interferometer. In addition, demonstrating the nonreciprocal effect as induced by varying Φ 1 − Φ 2 is a demonstration of the gauge potential for photons that is induced by the photon–phonon interactions. Demonstrating the photonic AB effect We demonstrate the photonic AB effect by measuring the effect of the phase Φ 1 − Φ 2 using the experimental set-up shown in Fig. 2 . The set-up consists of a Mach–Zehdner interferometer with two arms. The upper arm in Fig. 2 , referred below as the ‘reference arm’, consists of a retro-reflector mounted on a translation stage driven by a piezoelectric actuator. The phase that a photon accumulates as it passes through the reference arm can be adjusted by changing the position of the retro-reflector. The lower arm of the interferometer, referred below as the ‘AOM arm’, contains the acousto-optic crystals. We probe the transmission of the interferometer for light incident from either the left or the right. Since the experiments aim at detecting nonreciprocal response induced by the effective photonic gauge potential, we have constructed the experimental set-up such that the photons injected either from the left or from the right propagate through identical paths as they transmit through the interferometer. In the experiments, besides the first-order diffractions, the AOMs also generate weak zero-order and higher-order diffractions. The separation angle between two adjacent diffraction orders is ~0.5 degrees at the RF-driving frequency used in the experiments. To select the first-order diffracted beams, two spatial filters are used (More details in Methods). In the first set of experiments, we fix the phase Φ 1 – Φ 2 in the AOM arm by choosing a time delay of 5 ns for the RF signals that drive the two AOMs. For all the experiments, we use a modulation frequency of Ω /2 π =50 MHz. The 5 ns time delay here therefore corresponds to the phase Φ 1 – Φ 2 = π /2. We scan the phase delay of the reference arm by applying a sweep voltage to the piezoelectric actuator that controls the position of the retro-reflector. Shown in Fig. 3 are the measured transmission powers along the two directions when light is transmitted either from the left or the right. As expected, sinusoidal optical power variations are detected as the retro-reflector is scanned linearly with respect to time. We also note that for this case with Φ 1 – Φ 2 = π /2, the transmitted power from left to right has a reverse shape of that from right to left. This clearly demonstrates that the AOMs introduce nonreciprocal phase delays; that is, when a laser beam passes through the AOMs from left to right a π /2 phase is introduced, and when a laser beam propagates from right to left through the AOMs it acquires a − π /2 phase. 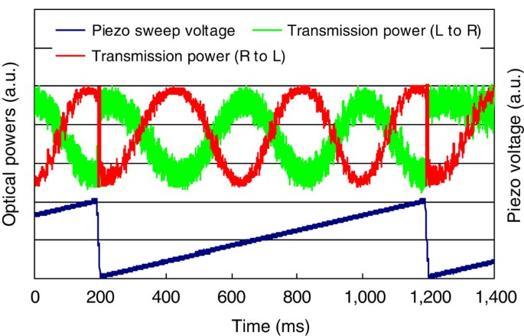Figure 3: Measured transmission optical powers in two opposite directions. The retro-reflector is scanned by applying a sweep voltage to the piezoelectric actuator. The AOM arm delay is set at 5 ns (that is,π/2 phase delay). The base lines for the optical power traces are shifted for illustration purpose. The experiments match well with the theoretical predictions. Figure 3: Measured transmission optical powers in two opposite directions. The retro-reflector is scanned by applying a sweep voltage to the piezoelectric actuator. The AOM arm delay is set at 5 ns (that is, π /2 phase delay). The base lines for the optical power traces are shifted for illustration purpose. The experiments match well with the theoretical predictions. Full size image In the second set of experiments, we then set the phase delay of the reference arm at π /2 by adjusting the retro-reflector’s position, and measure the transmission powers from the two directions as we vary the delay Φ 1 – Φ 2 through the AOM arm, as shown in Fig. 4 . For comparison purpose, the theoretically calculated curves for a period of 20 ns (the period of the AOM signals) are also plotted in Fig. 4 . It can be seen that the measured results are in reasonably good agreement with the predictions. We can see a contrast as large as 13 dB in the transmissions of the two directions has been achieved, indicating very strong nonreciprocal response from this system. The contrast can be further improved by matching the optical powers of the reference arm and the AOM arm of the interferometer through more precise alignment in experiments. The nonreciprocal sinusoidal oscillation of the transmission as a function of Φ 1 – Φ 2 is a direct demonstration of the photonic AB effect. 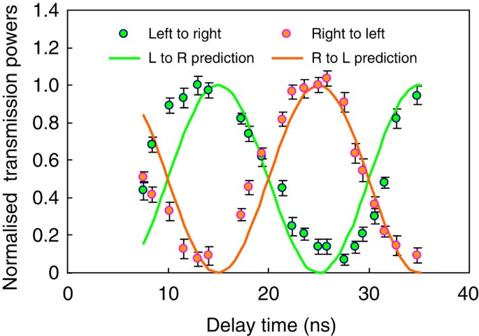Figure 4: Measured transmission optical powers in two opposite directions at different delay times (optical phases) introduced by the AOMs. The reference arm delay is set atπ/2. The periods of the optical power variations for both directions are close to 20 ns, which is the period of the RF-driving signals (50 MHz) used in our experiments. For each data point, 1,024 samples are collected and the standard derivations are used for plotting the error bars. Figure 4: Measured transmission optical powers in two opposite directions at different delay times (optical phases) introduced by the AOMs. The reference arm delay is set at π /2. The periods of the optical power variations for both directions are close to 20 ns, which is the period of the RF-driving signals (50 MHz) used in our experiments. For each data point, 1,024 samples are collected and the standard derivations are used for plotting the error bars. Full size image We utilize the photon–phonon interactions to introduce nonreciprocal phases for photons in the visible range, and observe experimentally a gauge potential for photons based on the photon–phonon interaction through the demonstration of a photonic AB effect. The results presented here point to new possibilities to control and manipulate photons by designing an effective gauge potential. We use bulk optics in our experiments to verify the principle of operation of the proposed scheme. The photon–phonon interactions can occur in different platforms, including waveguides and photonic crystals. Acousto-optic interaction of guided optical waves and surface acoustic waves in glass films on quartz substrates has been investigated since 1970s, and various thin-film acousto-optic technologies and devices have been developed and found wide applications [23] . More recently, stimulated Brillouin scattering, another form of photon–phonon interaction at tens of gigahertz frequencies, has been observed in photonic chips [24] and nanoscale silicon waveguides [25] . By incorporating the latest developments in photonics and integrated optics, the photon–phonon interaction scheme demonstrated in this work could be utilized to fabricate integrated photonic devices such as magnet-free on-chip isolators. Experimental methods Two identical He–Ne lasers with power outputs of 2 mW are used as the coherent light sources. For the left to right propagation, the laser beam is first split by a beam splitter (BS) into two beams. One of the two beams is reflected by a mirror, and then enters the phase shifter consisting of AOM1 and AOM2. Another beam, as a reference beam, passes through a delay line consisting of a retro-reflector (RR) and a pair of mirrors to generate phase delays to the reference beam. The interfering beams are combined at the second beam splitter/combiner (BS) and directed to a photo-detector through a flip mirror (FM). In the right to left propagation, the laser beams follow the reverse directions of the left to right propagation. By using two flip mirrors, we can switch between the two propagation directions. The material of the acousto-optic crystals is PbMoO 4 . The first-order diffraction efficiency of the AOMs is ~80% at a driving power of 1 W. The AOMs could also generate weak zero-order and higher-order diffractions. The separation angle between two adjacent diffraction orders is ~0.5 degrees at the RF-driving frequency used in the experiments. To select the first-order diffracted beams, two spatial filters (AP) are used. The RF signal generated by a signal generator (SG) is simultaneously fed into a power amplifier (A) for driving AOM1 and a programmable digital delay line (DL) that acts as an electronic phase shifter. The phase-shifted RF signal is amplified by a second power amplifier before feeding to AOM2. The frequency of the RF-driving signals is 50 MHz, giving a period of 20 ns. The increment of the programmable digital delay line is 0.25 ns. The phase delays between the two AOM-driving signals are monitored and measured by using a digital oscilloscope. The experimental set-up is built on an optical table to isolate the vibrations, and an enclosure covers the whole set-up to avoid the influence of air flows. Precise alignments of optics are needed for ensuring the two interferometers overlapped and exactly coaligned to each other. Careful adjustments of the AOM orientations are also necessary to balance the optical powers of the interfering beams for maximizing the fringe contrast. To test the left to right propagation, we set the flip mirror (FM) on the left side at ‘DOWN’ position and the flip mirror (FM) on the right side at ‘UP’ position, and vice versa for the right to left propagation. To account for the phase delays from the electronic delay circuit to the AOMs, the phase delays between the two AOM-driving signals are calibrated by connecting the RF signals from the BNC connectors at the AOMs to the digital oscilloscope with two identical cables. How to cite this article: Li, E. et al. Photonic Aharonov–Bohm effect in photon–phonon interactions. Nat. Commun. 5:3225 doi: 10.1038/ncomms4225 (2014).